The plastid ancestor originated among one of the major cyanobacterial lineages The primary endosymbiotic origin of chloroplasts is now well established but the identification of the present cyanobacteria most closely related to the plastid ancestor remains debated. We analyse the evolutionary trajectory of a subset of highly conserved cyanobacterial proteins (core) along the plastid lineage, those which were not lost after the endosymbiosis. We concatenate the sequences of 33 cyanobacterial core proteins that share a congruent evolutionary history, with their eukaryotic counterparts to reconstruct their phylogeny using sophisticated evolutionary models. We perform an independent reconstruction using concatenated 16S and 23S rRNA sequences. These complementary approaches converge to a plastid origin occurring during the divergence of one of the major cyanobacterial lineages that include N 2 -fixing filamentous cyanobacteria and species able to differentiate heterocysts. The appearance of free oxygen in the atmosphere results from an evolutionary biological breakthrough, and probably represents the most important biogeological event in Earth history. The innovation of oxygen-evolving photosynthesis occurred in precursors of cyanobacteria—a monophyletic group of microalgae recognized among prokaryotes by their ability to evolve oxygen. Cyanobacteria are also responsible for the spread of phototrophy among eukaryotic lineages. Many lines of evidence support that the (oxy)photosynthetic lifestyle of Archaeplastida (an evolutionary lineage grouping Glaucophyta, red and green algae, and green plants) derived from a common cyanobacterial ancestor that established a permanent endosymbiotic relationship with a mitochondriate ancestor. Some descendants of this primary endosymbiont underwent subsequent independent events (secondary and tertiary eukaryotic endosymbiosis), leading to the spread of oxygenic photosynthesis across an extremely diverse array of protists [1] , [2] , [3] , [4] , [5] , [6] , [7] . Cyanobacterial diversification was accompanied by one of the most outstanding increases in physiological and morphological complexity of the prokaryotic world [8] . Cyanobacteria were first subdivided into five taxonomic sections on the basis of morphological complexity and reproduction mode [8] . Although this complexity has been the driving force of classical cyanobacterial taxonomy, the recognition of polyphyly of most characters (muticellularity, nitrogen fixation, and baeocyte formation) rendered the assignment of phylogenetic groups necessary. Shih et al . [9] have generated a cyanobacterial species tree from a concatenation of 31 conserved proteins from 126 genomes, which defines 7 clades A to G [9] . In Fig. 1 of their paper, they show the non-univocal correspondence between the subclades or groups and the five previously defined morphological subsections for which no specific or unique genetic determinants underlying these major phenotypes could be retrieved. The candidate phylum of Melainabacteria appears to be the closest non-photosynthetic sibling to cyanobacteria [10] . Gloeobacter violaceus PCC 7421 and a reduced number of Synechococcus strains (Group G) are descendants of early and most probably extinct divergent lineages [5] , [11] , [12] . These were followed by divergence of groups F (which includes Pseudanabaena strains) and D (which includes Acaryochloris and Thermosynechococcus strains). Most extant cyanobacteria diversified from two major cyanobacterial lineages: (i) Group C, which includes Prochlorothrix sp., Prochlorococcus / Synechococus subclades and Leptolyngbya sp., and (ii) Group A and B, which include a great diversity of unicellular and multicellular strains, among which some are able to differentiate specific cells (heterocysts, hormogonia, akinetes and baeocytes) [9] . 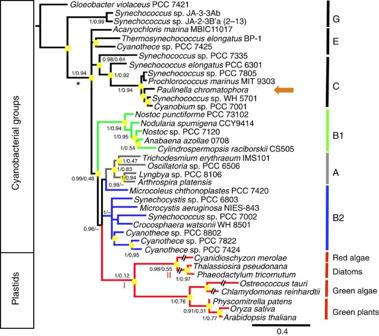Figure 1: Phylogenetic position of endosymbiotic events inferred from rRNA sequences. Phylogenetic relationships of cyanobacteria and plastids were inferred using model GTR+8Γ+CAT from alignments of concatenated sequences for small and large ribosomal subunits trimmed for reliable characters under default conditions. Yellow dots mark nodes conserved when data were trimmed under very stringent conditions. Phylogenetic subclades of cyanobacteria (A–G) are according to Shihet al.9. Red roman numbers indicate primary (I) and secondary (II) endosymbiotic events that gave rise to the Archaeplastida lineage from cyanobacteria, and the heterokont lineage from a red alga, respectively. The // symbols indicate plastid branches that have been graphically reduced to 10% of their original length. Scales represent genetic distances. Confidence values of branches supported with a posterior probability ≥95% are indicated together with their values after phylogenetic reconstruction of a multiple alignment trimmed under very stringent conditions (default/stringent). The arrow marks the independent primary endosymbiotic event from which the amoebaP. chromatophoraoriginates, and the asterisk (*) marks the plastid grafting point deduced from previous phylogenetic reconstructions4,9,13,16,22,25, and also observed using GTR+8Γ model. Figure 1: Phylogenetic position of endosymbiotic events inferred from rRNA sequences. Phylogenetic relationships of cyanobacteria and plastids were inferred using model GTR+8Γ+CAT from alignments of concatenated sequences for small and large ribosomal subunits trimmed for reliable characters under default conditions. Yellow dots mark nodes conserved when data were trimmed under very stringent conditions. Phylogenetic subclades of cyanobacteria (A–G) are according to Shih et al . [9] . Red roman numbers indicate primary (I) and secondary (II) endosymbiotic events that gave rise to the Archaeplastida lineage from cyanobacteria, and the heterokont lineage from a red alga, respectively. The // symbols indicate plastid branches that have been graphically reduced to 10% of their original length. Scales represent genetic distances. Confidence values of branches supported with a posterior probability ≥95% are indicated together with their values after phylogenetic reconstruction of a multiple alignment trimmed under very stringent conditions (default/stringent). The arrow marks the independent primary endosymbiotic event from which the amoeba P. chromatophora originates, and the asterisk (*) marks the plastid grafting point deduced from previous phylogenetic reconstructions [4] , [9] , [13] , [16] , [22] , [25] , and also observed using GTR+8Γ model. Full size image Molecular phylogenies using single or concatenated sequences converge to a monophyletic origin for plastids [4] , [9] , [13] , [14] , meaning that a single ancestral cyanobacterium underwent the successful primary event. However, the identification of the nearest current cyanobacterial species remains controversial (refs 1 , 9 , 13 , 15 and references therein for a recent analysis), hindering the inference for the morphological, biochemical and physiological characteristics of the ancestor. Most phylogenetic analyses based on 16S ribosomal RNA or single protein sequences showed that all the plastids group in a single radiation, and position the progenitor very close to the root (group G) of the cyanobacterial tree, before the divergence of the major lineages [4] , [5] . This ancient origin of plastids among the cyanobacterial radiation received support from phylogenetic reconstructions using concatenated protein and gene sequences of plants and cyanobacteria [9] , [13] , [15] , [16] . However, these single-gene phylogenetic and phylogenomic approaches are prone to important biases, as recently reviewed by Williams et al . [17] One approach to overcome pitfalls during reconstruction of ancient evolutionary events is to use refined models accounting for the phylogenetic landmarks that are diluted or buried (homoplasy) among a long and complex evolutionary history [18] . This must be accompanied by a strict selection of reliable phylomarkers among protein or DNA sequences that are resistant to horizontal gene transfer (HGT) and possess both strong evolutionary signals and a common phylogeny, as previously described [19] , [20] . Analysing the genetic makeup for 13 cyanobacterial genomes, Shi and Falkowski [20] identified 682 single-copy genes ubiquitous to all genomes and reported a subset of 323 sequences (the core) that possessed strong phylogenetic information and showed similar evolutionary trajectories as opposed to the other 359 sequences (the shell) that exhibited divergent phylogenies (that is, independent evolution and frequent transfers). Concatenation of core sequences allowed them to obtain a highly resolved and supported cyanobacterial tree. Given that these core genes had a similar evolutionary trajectory, our rationale was that if some homologous sequences are still retained in the descendants of the primary endosymbiont, the cyanobacterial core could be used for tracing the evolution of the plastid lineage among cyanobacteria. This approach should reduce the phylogenetic noise due to conflicting signals arising from the cyanobacterial sequences affected by site saturation, hidden paralogy and/or HGT events before endosymbiosis. Such conflicting signals may accumulate when the markers are identified by choosing homologous plastid sequences as seeds, as achieved in previous phylogenomic reconstructions [9] , [13] , [15] , [16] . Here we report on the evolutionary trajectory of cyanobacterial core genes once the last common ancestor of current cyanobacteria and plastids became an endosymbiont into a mitochondriate host. We identify and concatenate core sequences still present in cyanobacteria and photosynthetic eukaryotes for an accurate phylogenetic reconstruction using complex evolutionary models. The resulting phylogeny is congruent with an independent reconstruction using concatenated small and large rRNA sequences from the same species and previous physiological clues for the plastid origin. Our analysis places plastid origin among members of one of the major cyanobacterial lineages that includes filamentous N 2 -fixing cyanobacteria. The debate on plastid ancestor Single-loci phylogenetic reconstructions return an extremely large confidence set of trees [21] , supporting both a deep [22] and a recent [4] , [12] origin for plastids ( Supplementary Fig. 1 ). On the other hand, the phylogenomics results may be undermined by systematic errors if the phylogenetic reconstruction methods do not account for the complexity of the sequences (difference in evolutionary rates of sites and/or lineages) or if the concatenated data provide more phylogenetic noise (for example, hidden paralogy and HGT) than congruent phylogenetic information [17] , [19] , [20] , [23] . As a result, in such studies concatenated plastid sequences could group with ancient cyanobacteria (groups F and G) either as a consequence of long branching-attraction phenomenon [16] or of the heterogeneity of the evolutionary history of the concatenated sequences [18] . In contrast, a more recent origin—plastids diverging with Groups A and B—has been suggested based on phylogenetic analyses of concatenated rRNA sequences [12] , physiological data on starch storage [24] or protein similarity [1] , [25] . However, these analyses may also be biased as ribosomal sequences are susceptible of stochastic error [26] and evolutionary model misspecification ( Supplementary Fig. 1 ); common physiological traits can be acquired by convergence or retained by chance in different lineages and protein similarity can be enhanced by reduced evolutionary rates after divergence. Thus, further work is needed to accurately determine the origin of the plastid lineage. Phylogeny of concatenated 16S–23S rRNAs A thorough phylogenetic reconstruction using a concatenation of large and small rRNA sequences ( Supplementary Data 1 ) shows that the plastid lineage clusters with cyanobacterial groups A and B (posterior probability=0.99), as a sister group with group A and subgroup B2 (posterior probability=0.96) ( Fig. 1 ). In this analysis and in contrast to previous works [12] , [22] , we used an evolutionary model that accounts for heterogeneity among sites (CAT), allowing a good description of saturation and biochemical diversity of sequence alignments ( Table 1 ). Discrepancies with previous works could result from previous misspecification of the evolutionary model ( Supplementary Fig. 1 ). To further check the accuracy of the phylogenetic reconstruction, we increased the stringency for the selection of less-saturated characters in the multiple alignments ( Supplementary Data 2 ). As described for simulated data [27] , [28] , character trimming reduces confidence values for branches but increases the accuracy of phylogenetic reconstructions, that is, reduces the difference between the ‘true’ and the reconstructed trees. As expected from these previous works, confidence values for cluster support ≥0.95 (0.99 posterior probability on average) are reduced to an average of 0.74 after trimming. In spite of the increase in stringency, phylogenetic reconstruction recovered the monophyly of plastids as well as its clustering with groups A and B, but not as a sister of groups A and B2. This suggests that plastids arose during the diversification of the main groups. However, it does not end the current controversy on plastid origin, as the resulting topology differs from that obtained through previous phylogenomic approaches [9] , [13] , [15] , [16] , [25] . Table 1 Relevance of accounting for site heterogeneity during phylogenetic reconstructions. Full size table Phylogenomic of the core genes in photosynthetic eukaryotes We mined the complete sequences of cyanobacterial genomes and photosynthetic eukaryotes for the 323 cyanobacterial core sequences (as in May 2010, Supplementary Table 1 ). The number of sequences kept varies across photosynthetic eukaryotes with only 38 common to all photosynthetic eukaryotes ( Supplementary Data 3 ). Thus, only a few cyanobacterial core genes appear essential for intracellular lifestyle. To further test our first results, we added to the 13 analysed by Shi and Falkowski [20] 16 genomes chosen on the basis of their belonging to distant groups, genome size and evolutionary rate. To reconstruct the cyanobacterial/plastid evolutionary history, we started with only 68 (out of 323) cyanobacterial core genes (PCD data set, Supplementary Data 4 ), none being duplicated in the available cyanobacterial sequences (as May 2011) and all being present simultaneously in a diatom ( Phaeodactylum tricornutum ), a red alga ( Cyanidioschyzon merolae ) and a green plant ( Physcomitrella patens ). This data set was further reduced to 48 sequences (CyPlas data set, Supplementary Data 4 ), those for which protein trees were congruent ( P -value>0.05, Supplementary Data 4 ) with at least one of six topologies for the species tree ( Supplementary Fig. 2 and Supplementary Data 5–7 ); these topologies are likely to approach the evolutionary history of cyanobacteria. We further analysed the congruence of the CyPlas data set with five evolutionary scenarios: (i) the 16S–23S rRNA tree reconstructed using Phylobayes; (ii) two trees reconstructed from the concatenated CyPlas data set using both PhyML and Phylobayes; (iii) a consensus tree obtained with the 48 single-gene trees of the CyPlas data set; and (iv) a tailored tree in which plastids diverged together with heterocystous cyanobacteria as recently suggested [25] ( Fig. 2a–e and Supplementary Data 8–10 ). 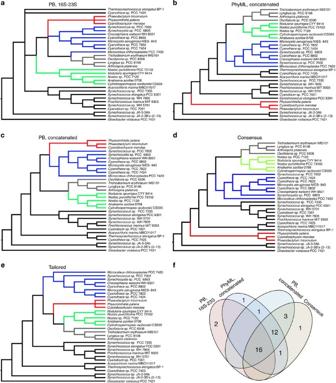Figure 2: Selection of phylomarkers for phylogeny of cyanobacteria and plastids. CyPlas data set (48 cyanobacterial sequences aligned with the corresponding homologous proteins from three photosynthetic eukaryotes) was checked for its congruence with the following evolutionary scenarios: (a) Phylobayes (PB) reconstruction of concatenated 16S–23S rRNAs sequences using the model GTR-8Γ-CAT; (b) PhyML and (c) Phylobayes reconstructions of concatenated CyPlas data set using models LG-16Γ and GTR-d-CAT, respectively; (d) a consensus tree of individual CyPlas data set phylogenies; as well as (e) a tailored tree to cluster plastid lineage with heterocystous cyanobacteria as recently suggested1. Red, grey, green and blue branches identify plastids, group A, subgroup B1 and subgroup B2 cyanobacterial lineages, respectively. (f) Venn diagram showing the distribution of the congruent genes among the phylogenies. Phylogenies based on protein sequences (Consensus, PhyML and Phylobayes) are the best guide trees for the common evolutionary history of individual gene trees, being in the confidence set ( P -value≥0.05) of 33 sequences ( Table 2 ). In fact, 28 of these genes were congruent simultaneously with topologies supporting an ancient origin of plastids (proposed by the PhyML and consensus trees) over a recent origin of plastids (proposed by Phylobayes tree), highlighting their limits to solve cyanobacteria–plastid phylogeny ( Fig. 2f ). Figure 2: Selection of phylomarkers for phylogeny of cyanobacteria and plastids. CyPlas data set (48 cyanobacterial sequences aligned with the corresponding homologous proteins from three photosynthetic eukaryotes) was checked for its congruence with the following evolutionary scenarios: ( a ) Phylobayes (PB) reconstruction of concatenated 16S–23S rRNAs sequences using the model GTR-8Γ-CAT; ( b ) PhyML and ( c ) Phylobayes reconstructions of concatenated CyPlas data set using models LG-16Γ and GTR-d-CAT, respectively; ( d ) a consensus tree of individual CyPlas data set phylogenies; as well as ( e ) a tailored tree to cluster plastid lineage with heterocystous cyanobacteria as recently suggested [1] . Red, grey, green and blue branches identify plastids, group A, subgroup B1 and subgroup B2 cyanobacterial lineages, respectively. ( f ) Venn diagram showing the distribution of the congruent genes among the phylogenies. Full size image Table 2 Set of 33 cyanobacterial core genes selected. Full size table The set of 33 sequences of plastids and cyanobacteria having a congruent evolutionary history ( Table 2 ) were concatenated for phylogenetic reconstructions ( Supplementary Data 11 ). In agreement with previously published analyses, maximum likelihood and Bayesian inference using LG+discrete gamma rate substitutions (Γ) evolutionary model supported with maximal statistical values (approximate Likelihood-Ratio Test (aLRT) and posterior probability=1) the basal emergence of plastids among the cyanobacterial tree ( Supplementary Fig. 3A ). However, this high statistical support does not necessarily ensure an accurate phylogenetic reconstruction if it is not supported by model assessment [18] , [29] . A posterior predictive analysis confirms that the PhyML topology that points to an ancient origin for plastids was the result of a model misspecification and that the LG+ Dirichlet (d)+CAT model, which accounts for heterogeneity across sites (CAT), is a good prediction of evolutionary history ( Supplementary Fig. 3C ). This model was further improved by accounting for heterogeneity over time (General-Time-Reversible model (GTR)+d+CAT model) without any change in the topology ( Fig. 3 ). The clustering of plastid lineage with groups A and B (posterior probability=0.99) is congruent with our previous reconstruction using ribosomal sequences ( Fig. 1 ). The distance from the plastid grafting point to the tips of heterocystous cyanobacteria appears as the shortest among the tree, in agreement with the remarkable similarity of the cyanobacterial proteins inherited by plants with those from heterocystous (Group B1) organisms [1] , [25] . The inclusion of Porphyra purpurea sequences in the data set reduces the number of available genes from 33 to 30 ( Supplementary Data 12 ). This does not alter the tree topology but increases to 0.99 the posterior probability for the monophyly of plastids ( Supplementary Fig. 4A ). In contrast, the additional inclusion of Cyanophora paradoxa and four cyanobacteria ( Gloeocapsa sp. PCC 7428, Rivularia sp. PCC 7116, Oscillatoria sp. PCC 6506 and Crinalium epipsammum PCC 9333) reduces the number of congruent genes to 18 ( Supplementary Data 13 ), which results in a reduction of branch support, whereas it maintains the Group A, B and plastid cluster ( Supplementary Fig. 4B ). These results thus point to the diversification of plastids within the major cyanobacterial lineages. 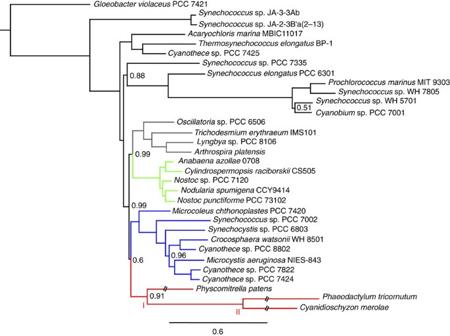Figure 3: Core phylogenomics converges on a recent origin for plastids. Phylobayes reconstruction of cyanobacteria and plastids inferred from alignments of 33 orthologous proteins concatenated and refined model GTR+d+CAT. Phylogenetic subclades of cyanobacteria (A–G) are according to Shihet al.9Red roman numbers indicate primary (I) and secondary (II) endosymbiotic events that gave rise to the Archaeplastida lineage from cyanobacteria, and the heterokont lineage from a red alga, respectively. The // symbols indicate plastid branches that have been graphically reduced to 10% of their original length. Scales represent genetic distances. Only posterior probabilities <1 are shown at nodes. Figure 3: Core phylogenomics converges on a recent origin for plastids. Phylobayes reconstruction of cyanobacteria and plastids inferred from alignments of 33 orthologous proteins concatenated and refined model GTR+d+CAT. Phylogenetic subclades of cyanobacteria (A–G) are according to Shih et al . [9] Red roman numbers indicate primary (I) and secondary (II) endosymbiotic events that gave rise to the Archaeplastida lineage from cyanobacteria, and the heterokont lineage from a red alga, respectively. The // symbols indicate plastid branches that have been graphically reduced to 10% of their original length. Scales represent genetic distances. Only posterior probabilities <1 are shown at nodes. Full size image Plastid origin versus cyanobacterial diversification The recent availability of genome sequences covering the wide cyanobacterial diversity [9] as well as of several photosynthetic eukaryotes allows to improve phylogeny by increasing the number and diversity of taxon sampling. Given the paucity of phylogenetically congruent proteins, we carried out a phylogenetic reconstruction using only concatenated rRNA sequences from 120 cyanobacteria, Paulinella chromatophora and 14 plastids ( Supplementary Fig. 5 and Supplementary Data 14 ). As the root of cyanobacteria has been recently questioned [30] , we included three diverse Melainabacteria (the closest related outgroup) [10] in the data set to root the phylogenetic tree constructed ( Supplementary Data 15 and 16 ). Reduction of data set complexity (number of sequences, redundancy, saturation and compositional heterogeneity) converges towards the clustering of plastid lineage with group A ( Fig. 4 , Supplementary Table 2 , Supplementary Figs 6 and 7 , and Supplementary Data 17–20 ). A recent phylogenetic reconstruction using concatenated protein-coding genes and refined methods ascribes this branching point to a compositional bias [15] . We observed however that the phylogenetic reconstruction after mitigation of compositional bias (from 13 to 2 s.d.) maintain plastid lineage as a sister of group A ( Supplementary Fig. 6 ). Noteworthy, after mitigation of compositional bias, the posterior probability of plastids as a sister of non-heterocystous filamentous N 2 -fixing cyanobacteria (members of family Oscillatoriaceae ) reaches a posterior probability of 0.9, as plastids cluster with group A with a bipartition frequency of 0.76, whereas they cluster with a Microcoleus strains with a bipartition frequency 0.14 ( Table 3 ). This is consistent with the hypothesis of heterocystous cyanobacteria as the more recent common ancestor of plastids [1] , as according to our phylogenetic analysis heterocystous cyanobacteria evolved from a non-heterocystous filamentous N 2 -fixing cyanobacteria of Group A or a Microcoleus related strains ( Figs 2 , 3 , 4 ). 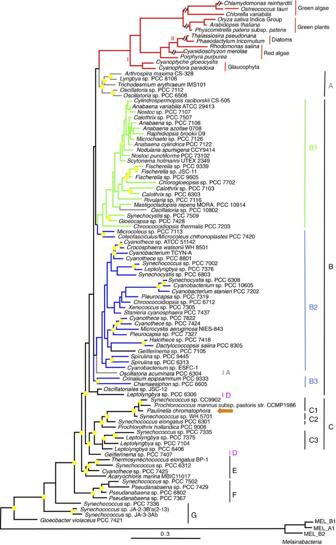Figure 4: Increasing the phylogenetic diversity of the rRNA data set places the plastid lineage as a sister of group A. Phylogenetic reconstruction (GTR+4Γ+CAT model) after removing redundancy (99 sequences and 1,029 variable sites remaining). As branch support is not reliable after the stringent trimming procedure27,28, accuracy of phylogenetic reconstruction can be inferred from the strong congruence of the cyanobacterial tree with a recent phylogenomic analysis9. Yellow dots mark matching clusters. Phylogenetic subclades of cyanobacteria (A–G) are according to Shihet al.9Red roman numbers indicate primary (I) and secondary (II) endosymbiotic events that gave rise to the Archaeplastida lineage from cyanobacteria and the heterokont lineage from a red alga, respectively. The // symbols indicate plastid branches that have been graphically reduced to 10% of their original length. Scales represent genetic distances. Figure 4: Increasing the phylogenetic diversity of the rRNA data set places the plastid lineage as a sister of group A. Phylogenetic reconstruction (GTR+4Γ+CAT model) after removing redundancy (99 sequences and 1,029 variable sites remaining). As branch support is not reliable after the stringent trimming procedure [27] , [28] , accuracy of phylogenetic reconstruction can be inferred from the strong congruence of the cyanobacterial tree with a recent phylogenomic analysis [9] . Yellow dots mark matching clusters. Phylogenetic subclades of cyanobacteria (A–G) are according to Shih et al . [9] Red roman numbers indicate primary (I) and secondary (II) endosymbiotic events that gave rise to the Archaeplastida lineage from cyanobacteria and the heterokont lineage from a red alga, respectively. The // symbols indicate plastid branches that have been graphically reduced to 10% of their original length. Scales represent genetic distances. Full size image Table 3 Mitigating compositional bias. Full size table The resulting rRNA tree supports the origin of plastids among already evolved cyanobacteria and fits the topology of the cyanobacterial groups of our phylogenomic tree: (i) it positions Gloeobacter at the root of the tree; (ii) Groups G, E and C diverge following the order described before; and (iii) it supports the divergence of plastids among already evolved cyanobacteria. Overall, our phylogenetic reconstructions using ribosomal and protein sequences were congruent. One important exception was the branching position of Microcoleus chthonoplastes PCC 7420, recently renamed Coleofasciculus chthonoplastes [31] . It clustered with subgroup B2 in protein phylogeny (in agreement with other phylogenomic reconstructions [13] , [25] but with group A in ribosomal phylogeny (in agreement with morphological and physiological data [31] , and exceptional domain acquisition of ValtRNA synthetases [32] ). Lodders et al . provided evidence that genetic recombination in natural populations of the cyanobacterium M. chthonoplastes frequently occurs [33] and that the nitrogenase cluster has been horizontally acquired [34] .This highlights the complex evolutionary history of this strain in which massive gene acquisitions have recently been reported [25] . Our results suggest that plastids arose during the diversification of groups A and B1 ( Fig. 4 ) that encompasses a majority of N 2 -fixing filamentous cyanobacteria; they are more closely related to group A, as they cluster with a relatively high support compared with well-described nodes. Thus, in contrast to the current dominant opinion, the plastid lineage probably has close relatives among extant cyanobacteria and it is not the sole survivor of an extinct lineage of cyanobacteria that diverged among groups G [13] , [15] and F [9] more than 2.5 Bya ago [3] , [5] . Current estimates date the group A and B1 diversification to some 1.75–2 Bya ago, and group A diversification to 1.5–1.75 Bya ago [5] , [12] , which is close to the date estimated for the primary endosymbiosis and for the last common ancestor of extant Archaeplastida (1.428–1.67 Bya) [3] , [35] , [36] , [37] and far from the Great Oxygenation Event (2.45–2.32 Bya) [5] . Our work accounts for previous discrepancies in the proposed phylogenies and gives support to a rather recent origin for the plastid lineage. It positions the last common ancestor of extant cyanobacteria and plastids after the diversification of clades A–B ( Figs 1 , 2 , 3 , 4 ), more probably as a sister group A ( Fig. 4 ). This diversification could have occurred 1.5–1.75 Bya ago, that is, after the Great Oxygenation Event [5] , [12] . Eukaryotes would thus not have been major factors in the early stages of the atmosphere oxygenation. Furthermore, the rise in atmospheric oxygen could have been the driving force that promoted some N 2 -fixing cyanobacteria to invade the microaerobic environment found in the cytosol of a mitochondriate phagotroph so as to protect their nitrogenase against O 2 inhibition. As feedback, the hosting cell may have benefitted from carbon and nitrogen-rich exudates from the endosymbiont. Although cyanobacterial endosymbioses are common in nature, for example, P. chromatophora or the diatom Rhopalodia gibba [2] being other examples, none of these more recent endosymbioses have however had the ecological success of the Archaeplastida primary plastid lineage or its secondary and tertiary plastid descendants. In addition, this work points to a set of core genes, and to a cluster of N 2 -fixing filamentous cyanobacteria (groups A and B1) on which future synthetic endosymbionts could be based. Experimental design Our phylogenomic experimental design involved: (i) a diversity-driven selection of cyanobacteria; (ii) the reconstruction of guide trees tracing the vertical evolution of this phylum; (iii) the identification of orthologous phylogenetic markers congruent to these trees; (iv) the addition to these markers of eukaryotic homologues of cyanobacterial origin; and (v) the phylogenetic reconstruction of cyanobacterial and plastid evolution using concatenated markers and refined evolutionary models. Taxonomic sampling Cyanobacteria were initially selected among 57 genomes available in 2010 on the basis of their position in a phylogenetic tree deduced from small subunit rRNA sequences; indeed this gene is a good diversity predictor of the universal gene core present in bacterial genomes [38] . As a rule, we identified the most divergent lineages from the root to the branch tips of the tree, and among these, the slowest evolving strains with the largest genomes ( Supplementary Table 1 ). We excluded closely related strains, as they add low genetic diversity while increasing the probability of incongruence by hidden/undetected HGT and biasing the heterogeneity of amino acids towards a given composition; this would have occurred if we had included all the marine Synechococcus and Prochlorococcus genomes [39] , [40] , [41] . The cyanobacterial data set was completed with photosynthetic eukaryotes for which the complete genome was available (May 2010). However, due to scarcity of orthologues for the reconstruction with concatenated sequences, this data set was reduced to three eukaryotes showing the highest diversity, slowest evolutionary rate and the largest number of cyanobacterial core genes in common: a diatom ( P. tricornutum ), a red alga ( C. merolae ) and a green plant ( P. patens ). The inclusion of a single green plant reduced the potential impact on incongruence test of duplications and hidden paralogy frequent in this lineage. Finally, as the position of the root of cyanobacteria was questioned during the work [30] , and the number of available genomes increased following a diversity-driven effort [9] , we expanded the taxon sampling to three diverse Melainabacteria [10] so as to root the phylogenetic tree, and to 120 cyanobacteria, P. chromatophora and 14 plastids from which a full set of small ( Supplementary Data 15 ) and large ( Supplementary Data 16 ) RNA gene sequences were available in June 2013 JGI-DOE [42] and SILVA Databases [43] . Data set selection, retrieval, concatenation and assessment Small and large ribosomal sequences were retrieved from JGI-DOE [42] and SILVA Databases, and aligned using SILVA tools [43] (bases remaining unaligned at the end were removed). BMGE [27] was used to remove gaps and constant positions from rRNA alignments and for selection of phylogenetic informative characters (-w 1 -h 1E-5:1 setting) under default (PAM100 matrix, -m DNAPAM100:2 -w 1 -g 0.0 -b 1 setting) or very stringent conditions (PAM1 matrix, -m DNAPAM1:2 -w 1 -g 0.0 -b 1 setting). A comparison of phylogenetic reconstructions using default and stringent conditions allowed us to estimate tree accuracy (more accurate under stringent conditions) and confidence values for branches (more reliable under default conditions) [27] , [28] . Constant sites were removed before phylogenetic reconstructions because it allows a better fit of models to data and reduces computing time. Eukaryotic proteins of cyanobacterial origin were identified after BLASTp searches [44] using the amino acid sequences from G. violaceus PCC 7421 ( Supplementary Data 2 as seed data set against Refseq-NCBI database [45] (Summer 2010), allowing 1,000–5,000 maximum target sequences. A eukaryotic top hit into the BLOSUM62 score range of cyanobacteria was the first evidence of a common origin. Blast results allowed us to ascertain the number of gene copies per cyanobacteria (using the Blast taxonomy report), the presence of eukaryotic counterparts and their evolutionary relationship with cyanobacteria (using Tree-blast phylogenetic reconstruction) either as a sister group or as originating from other bacteria. A second Blastp was performed to detect the absence/presence in photosynthetic eukaryotes by filtering for cyanobacteria and the selected eukaryotes. Selected protein sequences were retrieved and aligned (MAFFT [46] ) and translation start point reassigned (if required) using tBlastn [47] . Selection of reliable position (removing gaps and fastest evolving sites) were carried out using Gblock under default setting [48] . Guide trees To identify sequences orthologous to cyanobacterial genes, we used several guide trees that probably approximate the ‘real’ species tree. For the reconstruction of guide trees, we used two phylogenetic reconstruction approaches, PhyML 3.0 (ref. 49 ) and Phylobayes 3.3e [50] , and three different alignments: (i) small subunit rRNA sequences ( Supplementary Data 5 ), (ii) a concatenation of the large and small rRNA sequences ( Supplementary Data 6 ) and (iii) a concatenation of protein phylogenetic markers exhibiting a congruent evolutionary history [11] ( Supplementary Data 7 ). The latter was done in two steps [47] : we first concatenated Cicarelli’s sequences [11] to carry out a phylogenetic reconstruction using Phylobayes (GTR+4Γ+CAT). Approximately unbiased (AU) test [51] , [52] was used to select a subset of sequences congruent with the resulting topology. These 13 sequences were in turn concatenated ( Supplementary Data 7 ) and used for the reconstruction of the guide trees shown in Supplementary Fig. 2 . Evolutionary model selection and phylogenetic reconstruction We used the Akaike Information Criteria implemented in jModelTest 0.1 (ref. 53 ) and Prottest 2.4 (ref. 54 ) to select the best evolutionary models for the PhyML [49] reconstruction of DNA and protein sequence alignments, respectively. Model selection progressed in two steps. We first delimited the number of evolutionary models by selecting the best two models among 88 (jModelTest) or 14 (ProtTest) candidate models, and then we improved the model adjusting Γ discontinuous rates from 4 to 16. However, for the PhyML reconstruction of multiple alignments containing more than 90 sequences, we used the Bayesian Information Criteria and Model Averaged Phylogeny implemented in jModelTest 2.1.4 (ref. 55 ) to select the best evolutionary models among 1,624 available. Models were finally refined using Phylobayes 3.e to account for compositional heterogeneity across sites (CAT, 20 profiles) [29] and over time (GTR) [50] as well as rates across sites, following either a Dirichlet (d) process or discrete Γ distributions from 4 to 16 categories. To select the best evolutionary model among Bayesian reconstructions, we carried out a posterior predictive analysis of saturation (number of substitutions and level of homoplasy) and of the mean number of different amino acids per column [29] using the ppred programme implemented in Phylobayes. A consensus tree was obtained from trees sampled from the chain showing the best posterior predictions. Convergence of two chains was achieved using a parallelized version of phylobayes (MPI phylobayes [56] ) and was checked with the bpcomp programme, whereby convergence was reached if the maxdiff value of the four chains was ≤0.1. All Bayesian analyses were run at the University of Oslo’s Bioportal ( www.bioportal.uio.no ), Calendula (FCSCL, León, Spain) and Cipres Gateway [57] High Performance Computing Clusters. Finally, we evaluated the stability of the topology to variations in compositional heterogeneity (progressively suppressing sequences showing more than 3 or 2 s.d. of the mean) and taxon sampling ( Supplementary Data 20 ). Ppred programme implemented in Phylobayes was used to select sequences to mitigate compositional bias. Topology testing We used the Weighted Shimodaira–Hasegawa test implemented in CONSEL [51] to estimate the P -values of a set of topologies for a given alignment of sequences and its corresponding optimal evolutionary models ( Supplementary Data 3 ). Each of these models was used to calculate the likelihood per site of candidate trees (no more than 50 trees per run) using PhyML. Parameters and branch length (but not topology) were optimized and the branch support was not calculated. According to Shimodaira [52] , Weighted Shimodaira–Hasegawa test (WSH-test) is more adequate than AU test when several best trees (our six guide trees for cyanobacterial vertical evolution) are included in the set of candidate trees together with the optimal PhyML tree. To reduce sampling error, we increased ten times the number of replicates. We considered genes as orthologues if they had at least one guide tree topology in their confidence set of trees ( P -value>0.05). How to cite this article: Ochoa de Alda, J.A.G. et al . The plastid ancestor originated among one of the major cyanobacterial lineages. Nat. Commun. 5:4937 doi: 10.1038/ncomms5937 (2014).